Hypoxia-specific ultrasensitive detection of tumours and cancer cellsin vivo Highly sensitive and specific non-invasive molecular imaging methods are particularly desirable for the early detection of cancers. Here we report a near-infrared optical imaging probe highly specific to the hypoxic tumour microenvironment to detect tumour and cancer cells with the sensitivity to a few thousands cancer cells. This oxygen-sensitive, near-infrared emitting and water-soluble phosphorescent macromolecular probe can not only report the hypoxic tumour environment of various cancer models, including metastatic tumours in vivo , but can also detect a small amount of cancer cells before the formation of the tumour based on the increased oxygen consumption during cancer cell proliferation. Thus, the reported hypoxia-sensitive probe may offer an imaging tool for characterizing the tumour microenvironment in vivo , detecting cancer cells at a very early stage of tumour development and lymph node metastasis. Early detection plays a central role in improving the outcome of cancer treatment and increasing the overall survival. However, imaging the early stages of tumour formation and development in vivo remains a great challenge due to the limitations in the sensitivity of current molecular imaging probes, delivery of the probes and the interference of intrinsic background signals [1] , [2] . Thus, the development of effective imaging probes that can help visualize the tumour development, which spans from the abnormal proliferation of a few neoplastic cells to the formation and growth of a solid tumour, would impact the current strategies for early diagnosis. In addition, the ability to non-invasively image the early events of tumour formation will enable reporting cancer metastases and residual tumour cells after surgical treatment. Hypoxia, defined as oxygen-deprived condition, is a characteristic feature of the tumour microenvironment in most solid tumours due to the imbalance between new blood vessel formation and rapid proliferation of cancer cells [3] , [4] , [5] , [6] . Tumour hypoxia leads to an increased level of regulatory transcription factors such as hypoxia inducible factor 1α (HIF-1α) to upregulate the expression of genes associated with tumour initiation, malignant progression, metastasis and resistance to chemotherapy and radiotherapy [7] , [8] , [9] , [10] , [11] . Therefore, imaging hypoxic areas is of great interest for characterizing a tumour to determine the treatment strategy and can be potentially used to detect the early tumour formation and monitor the treatment response. Early reports on the development of non-invasive hypoxia imaging probes are typically based on nitroimidazole compounds that can be used for positron emission tomography imaging and magnetic resonance imaging [12] , [13] . However, the sensitivity of these probes is not sufficient as binding of the probes to hypoxic cells may require the oxygen concentration reaching an extremely low level [14] , [15] and the probes interacting with hypoxic cells for a significant period of time before being detected [16] . Furthermore, the binding of these probes to hypoxic cancer cells is also significantly impaired by the low pH of the tumour [17] , [18] . All of these limitations compromise the ability of these probes to detect hypoxia in the tumour. On the other hand, phosphorescent transition metal complexes have shown to be very effective in imaging and sensing the oxygen level in biological samples [19] , [20] , given the high sensitivity to oxygen, tunable excitation and emission wavelength and high luminescent quantum yields [21] , [22] . However, the phosphorescent transition metal imaging probes have poor biodistribution and pharmacokinetic profiles for tumour imaging due to non-specific uptake by normal tissues, binding to plasma proteins and rapid renal clearance, limiting their ability to differentiate hypoxic and normoxic conditions [23] . Moreover, these oxygen-sensitive probes are often water insoluble and have poor tissue penetration due to ultraviolet–visible emitting, preventing their application to hypoxia imaging in vivo [24] , [25] , [26] , [27] . In this work, we are reporting a water-soluble and stable phosphorescent macromolecular probe for hypoxia imaging with high sensitivity and specificity. This poly( N -vinylpyrrolidone) (PVP)-conjugated iridium (III) complex probe ( Fig. 1a ) is an oxygen-sensitive, near-infrared (NIR)-emitting macromolecule consisting of two key functional components. The first component is the iridium (III) complex containing a large conjugated ligand that extends phosphorescence emission spectra to the NIR region, allowing light penetration for deep-tissue imaging. The phosphorescence emission of the iridium (III) complex is quenched by oxygen in normal tissues but turns on at the reduced oxygen level in tumour tissues, providing hypoxia specificity of imaging with minimal background interference. The second component is the hydrophilic PVP polymer that improves tumour retention time via enhanced permeation and retention effect. PVP was originally developed as a plasma substitute [28] , [29] . Currently, it is widely used as a retarding agent in medicine to improve the plasma half-life of drugs [30] . Compared with polyethylene glycol, PVP does not trigger accelerated blood clearance phenomenon, which means the plasma concentration and residue time of PVP do not show significant decrease when it is repeatedly injected [31] . Besides, PVP is also more easily functionalized for further applications. Thus, the terminal group of the PVP chain can be linked to an internal standard (‘R’ group in Fig. 1a ), allowing for ratiometric measurement of the probe. Prolongation of action time offered by PVP allows for continuously monitoring tumour hypoxia to evaluate longitudinal and dynamic change in the tumour microenvironment. Here we investigate the capability and sensitivity of this probe for hypoxia imaging in vitro and in vivo using various cell lines and tumour models, including a metastatic tumour model. Our results show that the new probe provides non-invasive hypoxia-based ultrasensitive detection and differentiation of cancer cells in vivo even before the formation of a solid tumour. 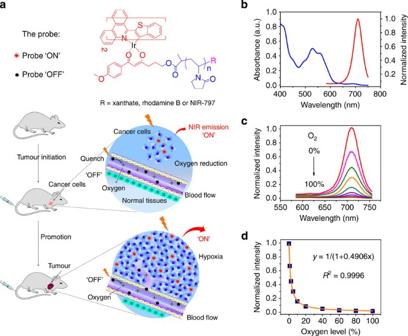Figure 1: Chemical structure and optical properties of the probe. (a) The chemical structure of the probe and a schematic of tumour/cancer cell detection with the probe. The phosphorescence emission of the probe is quenched by oxygen in the vessels and normal tissues. In contrast, the probe emits strong NIR phosphorescence when meeting cancer cells and tumours. (b) Ultraviolet–visible absorption (blue line) and emission (red line) spectra of Ir-PVP in deaerated aqueous solution at room temperature. (c) Emission spectra of Ir-PVP under increasing oxygen levels (0, 1, 2.5, 5, 10, 20, 40, 60, 80 and 100%). Excitation: 560 nm. (d) The decay curve of peak phosphorescent intensity of Ir-PVP over the increase of oxygen level (0, 1, 2.5, 5, 10, 20, 40, 60, 80 and 100%). Figure 1: Chemical structure and optical properties of the probe. ( a ) The chemical structure of the probe and a schematic of tumour/cancer cell detection with the probe. The phosphorescence emission of the probe is quenched by oxygen in the vessels and normal tissues. In contrast, the probe emits strong NIR phosphorescence when meeting cancer cells and tumours. ( b ) Ultraviolet–visible absorption (blue line) and emission (red line) spectra of Ir-PVP in deaerated aqueous solution at room temperature. ( c ) Emission spectra of Ir-PVP under increasing oxygen levels (0, 1, 2.5, 5, 10, 20, 40, 60, 80 and 100%). Excitation: 560 nm. ( d ) The decay curve of peak phosphorescent intensity of Ir-PVP over the increase of oxygen level (0, 1, 2.5, 5, 10, 20, 40, 60, 80 and 100%). Full size image Synthesis and characterization of the probe The probe, Ir-PVP, was synthesized following the scheme shown in Supplementary Fig. 1 . For ratiometric measurements, Ir-PVP probe linked with Rhodamine B (Ir-PVP-RhB) or NIR-797 (Ir-PVP-N797) was also prepared based on the chemical reactions on the terminal group of PVP ( Supplementary Figs 2 and 3 ). For comparison, a small-molecular iridium (III) complex without PVP chain (Ir-OH) was synthesized ( Supplementary Fig. 4 ). The ultraviolet absorption and photoluminescence spectra of Ir-PVP in deaerated aqueous solution show that Ir-PVP has two intense absorption peaks at 530 and 560 nm as well as a strong phosphorescence emission peak at 710 nm when excited at 560 nm ( Fig. 1b ). The phosphorescence quantum yield of Ir-PVP is 0.15 in the Ar-saturated aqueous solution with a lifetime of about 1.0 μs in the air-equilibrated aqueous solution. The phosphorescence emission intensity of Ir-PVP in the aqueous solution increased non-linearly as the level of oxygen decreased ( Fig. 1c ). The ratio of phosphorescence intensities in oxygen-free to oxygen-saturated Ir-PVP aqueous solutions is as high as 62. The decay curve of phosphorescent intensity of the peak as a function of the oxygen level reveals that the probe is especially sensitive to oxygen under lower oxygen levels (<5%), where a small decrease of the oxygen level leads to a sharp increase in the phosphorescent intensity of the probe ( Fig. 1d ). For instance, a 1% decrease in oxygen level induced 50% increase in probe intensity, making the probe particularly suitable for hypoxia imaging in the physiological conditions. Compared with a widely used and commercially available intracellular oxygen probe (Mito-ID intracellular O 2 probe, Enzo Life Sciences), Ir-PVP exhibited much higher oxygen sensitivity ( Supplementary Fig. 5 ). It should also be mentioned that the phosphorescent emission of Ir-PVP remains constant in a broad pH range of 2.0–8.0, thus it is applicable in the acidic conditions ( Supplementary Fig. 6 ). This is particularly important for the imaging of tumour hypoxia since most solid tumour tissue and environment are acidic. We also estimated the tissue penetration depth of the optical signal from Ir-PVP to be 9 mm ( Supplementary Fig. 7 ). In vitro imaging of cell response to hypoxia To test Ir-PVP for the imaging of cells in hypoxia, human neuroblastoma SH-SY5Y cells were incubated with Ir-PVP in the presence of 0, 10 and 21% of oxygen. It was found that under culture conditions the cell-bound probes did not emit phosphorescence when exposed to the atmospheric oxygen partial pressure, that is, 21% O 2 ( Fig. 2a ). When the O 2 concentration decreased to 0%, the probes bound to cells started to emit intense phosphorescence. Similar results were observed in murine hepatic cancer cell line H22 ( Fig. 2a ). Thus, Ir-PVP exhibits remarkable hypoxia-dependent phosphorescence sensitivity for cell imaging. 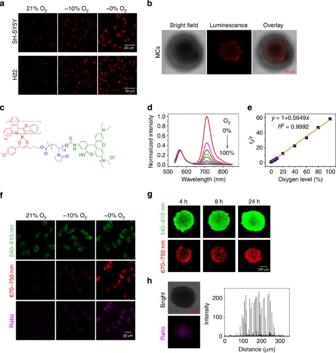Figure 2: Imaging of cancer cell hypoxiain vitrowith the Ir-PVP probe. (a) Confocal luminescence images of living SH-SY5Y cells and H22 cells treated with Ir-PVP (0.2 mg ml−1) and incubated at three different oxygen levels (21, ~10 and ~0%). (b) Confocal luminescence images of SH-SY5Y MCs after incubation with Ir-PVP (0.2 mg ml−1) for 8 h. (c) Chemical structure of Ir-PVP-RhB. (d) Emission spectra of Ir-PVP-RhB under increasing oxygen levels (0, 2.5, 5, 7.5, 10, 20, 40, 60, 80 and 100%). Excitation: 510 nm. (e) The linear relationship betweenr0/rand the oxygen level. (f) Confocal luminescence images of SH-SY5Y cells treated with Ir-PVP-RhB (0.2 mg ml−1) and incubated at different oxygen levels. The signals were received in two channels (540–610 nm and 670–750 nm) with a single excitation at 514 nm. (g) Confocal luminescence images of SH-SY5Y MCs after incubation with Ir-PVP-RhB (0.2 mg ml−1) for different times. (h) Left: bright-field image of MCs and the image displaying the ratio (purple) between the signal of Ir and RhB moieties at the incubation time of 24 h. Right: the signal intensity profile corresponding to the map of signal ratio (left) showing the quantitative and spatial distribution of hypoxia in the selected cross-section of the MCs. The red arrow in the bright-field image shows the location of selected cross-section. Figure 2: Imaging of cancer cell hypoxia in vitro with the Ir-PVP probe. ( a ) Confocal luminescence images of living SH-SY5Y cells and H22 cells treated with Ir-PVP (0.2 mg ml −1 ) and incubated at three different oxygen levels (21, ~10 and ~0%). ( b ) Confocal luminescence images of SH-SY5Y MCs after incubation with Ir-PVP (0.2 mg ml −1 ) for 8 h. ( c ) Chemical structure of Ir-PVP-RhB. ( d ) Emission spectra of Ir-PVP-RhB under increasing oxygen levels (0, 2.5, 5, 7.5, 10, 20, 40, 60, 80 and 100%). Excitation: 510 nm. ( e ) The linear relationship between r 0 / r and the oxygen level. ( f ) Confocal luminescence images of SH-SY5Y cells treated with Ir-PVP-RhB (0.2 mg ml −1 ) and incubated at different oxygen levels. The signals were received in two channels (540–610 nm and 670–750 nm) with a single excitation at 514 nm. ( g ) Confocal luminescence images of SH-SY5Y MCs after incubation with Ir-PVP-RhB (0.2 mg ml −1 ) for different times. ( h ) Left: bright-field image of MCs and the image displaying the ratio (purple) between the signal of Ir and RhB moieties at the incubation time of 24 h. Right: the signal intensity profile corresponding to the map of signal ratio (left) showing the quantitative and spatial distribution of hypoxia in the selected cross-section of the MCs. The red arrow in the bright-field image shows the location of selected cross-section. Full size image Since multicellular spheroids (MCs) represent more closely the heterogeneity of the tumour microenvironment with a hypoxic core and normoxic surface [32] , [33] compared with traditional monolayer cell cultures, we incubated SH-SY5Y MCs with Ir-PVP. The strong phosphorescence signal of Ir-PVP was observed in the core of spheroids, while almost no signal was detected on the surface of spheroids ( Fig. 2b ), suggesting that Ir-PVP is sensitive enough to distinguish the hypoxic core and the normoxic surface of the MCs. Ratiometric measurement of hypoxia in vitro To evaluate the capability of quantitative assessment of hypoxia, ratiometric measurement was performed using the Ir-PVP-RhB ( Fig. 2c ). On excitation at 510 nm, Ir-PVP-RhB exhibits two emission peaks at 565 and 710 nm ( Fig. 2d ). The 710-nm emission from the iridium complex moiety (Ir moiety) is responsive to the change in oxygen level, while the 565-nm emission from the Rhodamine B moiety (RhB moiety) remains stable, thus it can be used as an internal standard of the probe concentration. Furthermore, the ratio (represented as r ) between the peak intensities of 710 and 565 nm corresponds to the oxygen level and is independent of the probe concentration. As shown in Fig. 2e , there is a linear relationship between r 0 / r and the oxygen level (where r 0 represents the ratio at 0% O 2 ). These results suggest that the quantitative assessment of hypoxia with the reported probe is feasible. Ir-PVP-RhB was then used to measure hypoxia in SH-SY5Y cells ( Fig. 2f ). With the decrease of the oxygen level, the signal from the RhB moiety (540–610 nm, green) showed almost no change, while the signal from the Ir moiety (670–750 nm, red) dramatically increased. The ratio (purple) between the latter and the former thus allows us to report the level of hypoxia. The spatial distribution and heterogeneity of hypoxic conditions in SH-SY5Y MCs were also measured using Ir-PVP-RhB ( Fig. 2g ). The gradual change of the signal from the RhB moiety (green) and Ir moiety (red) showed the depth and time-dependent penetration of the probe in the MCs. With prolonged incubation time, the probe reached further into the centre of the MCs. The map of the signal ratio (purple) between Ir and RhB moieties thus provides the quantitative and spatial distribution of hypoxic condition in the MCs ( Fig. 2h ). The signal profile from a cross-section of a MC ( Fig. 2h ) further demonstrates the capability and sensitivity of the probe in sensing the range and level of hypoxia conditions. Notably, we observed that the hypoxia signal is detected starting from about 100 μm from the edge, which is consistent with the result reported in the literature [15] . In vivo imaging of tumour hypoxia with Ir-PVP probe To examine the ability of Ir-PVP in the imaging of tumour hypoxia in vivo , the mice bearing subcutaneously implanted tumours grown from murine hepatoma cell line H22 were administered with intravenous (i.v.) injection of Ir-PVP (40 mg kg −1 ) and scanned at different time points after injection. As shown in Fig. 3a , the phosphorescence signal of the probe was exclusively observed in the tumour region without background signal during 1 to 120 h post injection. The photon counts s −1 measured in the tumour region at different time points ( Fig. 3b ) revealed that the phosphorescence intensity in the tumour region increased rapidly after the injection of the probe. It reached a maximum level at 8 h post injection, followed by a gradual decrease from 8 to 120 h post injection. 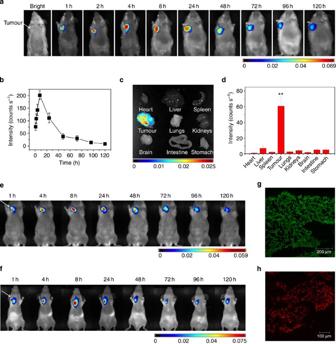Figure 3: Imaging of tumour hypoxiain vivowith Ir-PVP probe. (a) Whole-body optical imaging of ICR mice bearing subcutaneously implanted H22 tumour in the armpit after i.v. injection of Ir-PVP. (b) The photon counts detected per second in the tumour region at different time points after i.v. injection of Ir-PVP. The results are presented as the mean±s.d. (n=5). (c) The major organs of tumour-bearing mice were isolated and immediately imaged at 120 h after i.v. injection of Ir-PVP. (d) Signal intensities of Ir-PVP from different organs at 120 h post injection. The results are presented as the mean±s.d. (n=5). **P<0.01, in comparison between the tumour and other normal organs by a one-way analysis of variance (ANOVA). (e) Whole-body optical imaging of ICR mice subcutaneously implanted with 4T1 tumour in the armpit after i.v. injection of Ir-PVP. (f) Whole-body optical imaging of BALB/c nude mice subcutaneously implanted with HeLa tumour in the armpit after i.v. injection of Ir-PVP. (g,h) Frozen sections of the tumour were stained with HIF-1α antibody (g, green fluorescence) and pimonidazole antibody (h, red fluorescence). Figure 3: Imaging of tumour hypoxia in vivo with Ir-PVP probe. ( a ) Whole-body optical imaging of ICR mice bearing subcutaneously implanted H22 tumour in the armpit after i.v. injection of Ir-PVP. ( b ) The photon counts detected per second in the tumour region at different time points after i.v. injection of Ir-PVP. The results are presented as the mean±s.d. ( n =5). ( c ) The major organs of tumour-bearing mice were isolated and immediately imaged at 120 h after i.v. injection of Ir-PVP. ( d ) Signal intensities of Ir-PVP from different organs at 120 h post injection. The results are presented as the mean±s.d. ( n =5). ** P <0.01, in comparison between the tumour and other normal organs by a one-way analysis of variance (ANOVA). ( e ) Whole-body optical imaging of ICR mice subcutaneously implanted with 4T1 tumour in the armpit after i.v. injection of Ir-PVP. ( f ) Whole-body optical imaging of BALB/c nude mice subcutaneously implanted with HeLa tumour in the armpit after i.v. injection of Ir-PVP. ( g , h ) Frozen sections of the tumour were stained with HIF-1α antibody ( g , green fluorescence) and pimonidazole antibody ( h , red fluorescence). Full size image To confirm that the phosphorescence signal was from the probe accumulated in the tumour, we recorded ex vivo phosphorescence images of tumour and normal organs collected immediately after killing the mice at 120 h post injection. Consistent with the results observed in vivo , only the tumour yielded a strong phosphorescence signal ( Fig. 3c ). The photon counts s −1 measured from the tumour were at least 10 times higher than the normal organs ( Fig. 3d ). The ability of the probe to sense hypoxia in vivo was further demonstrated in the imaging of mice bearing with other tumour types, including mouse mammary carcinoma 4T1 cell line ( Fig. 3e ) and human epithelial carcinoma HeLa cell line ( Fig. 3f ), suggesting the robustness and broad applicability of the probe. Immunostaining for endogenous markers of hypoxia with HIF-1α antibody and pimonidazole antibody confirmed that the tumours were hypoxic with high levels of HIF-1α ( Fig. 3g,h and Supplementary Fig. 8 ). The emergence and increase of the signal from the probe thus reports the presence and conditions of hypoxic microenvironment in tumours. To further investigate and confirm hypoxia-specific tumour detection with the reported probe, we turned to Ir-PVP probe linked with a NIR dye NIR-797 (Ir-PVP-N797) ( Fig. 4a ). Ir moiety (710 nm emission) of Ir-PVP-N797 remains to be highly sensitive to oxygen level, while the NIR-797 moiety (825 nm emission) is insensitive to oxygen ( Fig. 4b ). Therefore, the signal from the NIR-797 moiety can be used as an internal standard to assess the probe concentration non-invasively in vivo . 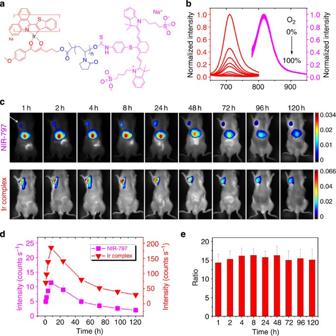Figure 4: Imaging of tumour hypoxiain vivowith Ir-PVP-N797. (a) Chemical structure of Ir-PVP-N797. (b) Emission spectra of Ir-PVP-N797 under increasing oxygen levels (0, 2.5, 5, 7.5, 10, 20, 40, 60, 80 and 100%). The 710-nm emission (red) is excited at 560 nm and the 825-nm emission (purple) is excited at 750 nm. (c) Whole-body optical images of ICR mice bearing subcutaneously implanted H22 tumours in the armpit after i.v. injection of Ir-PVP-N797 (40 mg kg−1). (d) The averaged signal intensities of Ir moiety (red) and NIR-797 moiety (purple) in the tumours at different time points after i.v. injection of Ir-PVP-N797. The results are presented as the mean±s.d. (n=5). (e) The ratio between the signal intensities of Ir moiety and NIR-797 moiety at different time points after i.v. injection of Ir-PVP-N797. The results are presented as the mean±s.d. (n=5). Figure 4: Imaging of tumour hypoxia in vivo with Ir-PVP-N797. ( a ) Chemical structure of Ir-PVP-N797. ( b ) Emission spectra of Ir-PVP-N797 under increasing oxygen levels (0, 2.5, 5, 7.5, 10, 20, 40, 60, 80 and 100%). The 710-nm emission (red) is excited at 560 nm and the 825-nm emission (purple) is excited at 750 nm. ( c ) Whole-body optical images of ICR mice bearing subcutaneously implanted H22 tumours in the armpit after i.v. injection of Ir-PVP-N797 (40 mg kg −1 ). ( d ) The averaged signal intensities of Ir moiety (red) and NIR-797 moiety (purple) in the tumours at different time points after i.v. injection of Ir-PVP-N797. The results are presented as the mean±s.d. ( n =5). ( e ) The ratio between the signal intensities of Ir moiety and NIR-797 moiety at different time points after i.v. injection of Ir-PVP-N797. The results are presented as the mean±s.d. ( n =5). Full size image Whole-body imaging of mice bearing subcutaneously implanted H22 tumours with signal from the NIR-797 moiety showed that the probe was mainly taken up by the liver in addition to accumulation in the tumour ( Fig. 4c ). However, imaging with phosphorescence signal from the Ir moiety showed that the signal from the tumour was outstanding with minimal background signals in normal tissue and organs even though there was a significant liver accumulation of the probe as shown in NIR imaging using the NIR-797 moiety ( Fig. 4c ). Measuring the intensities of the Ir moiety and NIR-797 moiety and calculating their ratios then allows for monitoring tumour hypoxia as well as probe distribution over time up ( Fig. 4d,e ). Since normal liver is highly vascularized with proper sufficient blood and oxygen supply compared with the highly hypoxic tumour, the increased phosphorescence signal in the tumour in contrast to the attenuation of phosphorescence signal in the liver supports that the probe is highly hypoxia specific with low interference from normal physiological conditions. We believe that reducing the off-target and non-specific background is critical to the sensitivity and specificity of the tumour detection, especially when the tumour-localized delivery of a probe reaches its threshold. 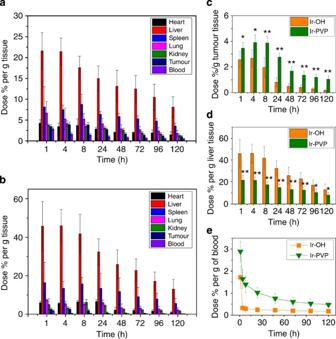Figure 5: Biodistribution of Ir-PVP and Ir-OH in ICR mice bearing H22 tumours. (a,b) Biodistribution of Ir-PVP (a) and Ir-OH (b) in different organs at various time points after i.v. injection of the probes. The values were presented as the percentage of injected dose per g of collected organ and based on five mice per group. (c,d) The concentrations of Ir-OH and Ir-PVP in the tumour (c) and liver (d) of the mice at various time points after i.v. injection of the probes. The results are presented as the mean±s.d. (n=5). *P<0.05 and **P<0.01, in comparison of the concentrations of Ir-PVP and Ir-OH using a two-sample Student’st-test. (e) Time-dependent blood clearance profiles of Ir-OH and Ir-PVP measured in the mice. Biodistribution of the probes in vivo Figure 5a,b shows the biodistributions of Ir-PVP and Ir-OH (the iridium (III) complex without PVP chain) in tissues, organs and blood of ICR mice bearing subcutaneously implanted H22 tumours. Ir-PVP exhibits significantly higher accumulation in the tumour compared with Ir-OH ( Fig. 5c ). For instance, the averaged Ir concentration in the tumour is 2.0% of the injected dose in per g of tumour tissue for Ir-OH at 1 h post injection, while the averaged Ir concentration in the tumour is 3.9% at the same time point for Ir-PVP. At 24 h post injection, the averaged Ir concentration reduced to 0.8% for Ir-OH compared with 2.8% for Ir-PVP. Meanwhile, the liver uptake of Ir-PVP is significantly lower than that of Ir-OH ( Fig. 5d ). At 1 h post injection, the averaged Ir concentration in the liver is 45.7% of the injected dose in per g of liver tissue for Ir-OH versus 21.5% for Ir-PVP. In addition, Ir-PVP shows a longer blood circulation time over Ir-OH ( Fig. 5e ). The blood half-life for Ir-PVP is 1.1 versus 0.4 h for Ir-OH. The lower liver uptake and longer blood circulation time of Ir-PVP are ascribed to its weaker serum albumin-binding ability than Ir-OH as determined by isothermal titration calorimetry ( Supplementary Fig. 9 ). The binding constant ( K ) of the probe to bovine serum albumin is 5.18 × 10 5 M −1 for Ir-PVP versus 9.41 × 10 6 M −1 for Ir-OH. The longer blood circulation time and reduced non-specific uptake of Ir-PVP should facilitate the higher tumour accumulation of the probe. These results suggest that the PVP chain of the probe plays a very important role in improving tumour accumulation and retention and prolonging the action time of the probe. Figure 5: Biodistribution of Ir-PVP and Ir-OH in ICR mice bearing H22 tumours. ( a , b ) Biodistribution of Ir-PVP ( a ) and Ir-OH ( b ) in different organs at various time points after i.v. injection of the probes. The values were presented as the percentage of injected dose per g of collected organ and based on five mice per group. ( c , d ) The concentrations of Ir-OH and Ir-PVP in the tumour ( c ) and liver ( d ) of the mice at various time points after i.v. injection of the probes. The results are presented as the mean±s.d. ( n =5). * P <0.05 and ** P <0.01, in comparison of the concentrations of Ir-PVP and Ir-OH using a two-sample Student’s t -test. ( e ) Time-dependent blood clearance profiles of Ir-OH and Ir-PVP measured in the mice. Full size image Biocompatibility and toxicity evaluation of the probe The biocompatibility of Ir-PVP was evaluated by its effect on the apoptosis and necrosis of SH-SY5Y cells. The early/late apoptosis and necrosis were stained with annexin V-FITC and propidium iodide and measured by flow cytometry ( Supplementary Fig. 10 ). Ir-PVP did not induce significant apoptosis or necrosis compared with the control at doses up to 1.6 mg ml −1 . The phototoxicity test revealed that the production of reactive oxygen species by Ir-PVP (1.6 mg ml −1 ) in SH-SY5Y cells was negligible under irradiation by 595 nm light source (40 J cm −2 ) and cell viability remained very high (>90%) after irradiation ( Supplementary Fig. 11 ). We further examined the blood coagulation behaviour and serum biochemistry of Ir-PVP in mice after the administration of the probe. Fibrinogen, prothrombin time and activated partial thromboplastin time showed no statistically significant differences between the probe treatment and control groups, indicating negligible effect of Ir-PVP on blood coagulation ( Supplementary Fig. 12 ). The liver function indexes, including alanine aminotransferase, aspartate aminotransferase and total bilirubin, and kidney function indexes, including blood urea nitrogen, creatinine and urea tests, appeared at normal ranges, demonstrating no hepatic dysfunction or renal toxicity ( Supplementary Fig. 13 ). Histopathology examination showed that the major organs, such as heart, liver, spleen, kidney and lung, retained similar morphologies 7 days after injection of Ir-PVP, compared with the control group ( Supplementary Fig. 14 ), indicating no detectable side effect of the probe. These results suggest that Ir-PVP is highly biocompatible. Detection of tumour cell metastasis in lymph nodes with Ir-PVP Given the high sensitivity and specificity of hypoxia imaging with Ir-PVP probe, we further investigated the capability of the reported probe in detecting lymph node metastasis. The mice bearing 4T1 tumours in the right paw that develop lymph node metastasis [34] were imaged after footpad injection of the probe from the right paw (8 mg kg −1 ). As shown in Fig. 6a , strong phosphorescence signals were observed not only in the primary tumour grown in the right paw but also in the inguinal lymph node of the tumour-bearing mice. The ex vivo examination revealed that the inguinal lymph node of the tumour-bearing mice was noticeably swollen and emitted a much stronger probe signal than the lymph node from normal mice ( Fig. 6b ). Haematoxylin and eosin-stained sections of the primary tumours and the inguinal lymph nodes collected from the tumour-bearing mice confirmed the presence of metastatic tumour cells ( Fig. 6c,d ). Furthermore, both primary tumour and lymph node metastases were found to be hypoxic based on the positive staining with HIF-1α antibody ( Fig. 6e,f ) and pimonidazole ( Fig. 6g,h ). These results show that the probe is not only very effective in the detection of primary tumour but also in the detection of lymph node metastasis. 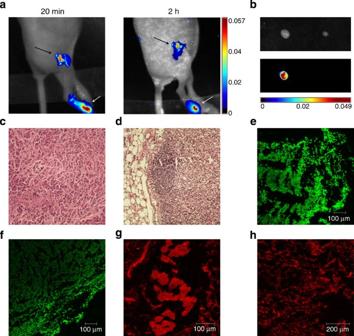Figure 6: Hypoxia-based detection of lymph node metastasis with Ir-PVP. (a) Optical images of ICR mice bearing 4T1 tumours in the paws show the hypoxic signals in the lymph nodes due to cancer cells metastasized to the nodes. Ir-PVP was administered through footpad injection in the right paw. The black arrows point to the area with lymph node metastases and the white arrows point to the primary tumour in the paw. (b) Bright and luminescent image of metastatic lymph node (left) and normal lymph node (right) 2 h after footpad injection of Ir-PVP in the right paw. (c,d) Haematoxylin and eosin-stained slices (× 200) of primary tumour (c) and lymph node metastases (d). (e,f) Frozen sections of the primary tumour (e) and lymph node with metastasis (f) were stained with HIF-1α antibody (green fluorescence). (g,h) Frozen sections of the primary tumour (g) and lymph node with metastasis (h) were stained with pimonidazole antibody (red fluorescence). Figure 6: Hypoxia-based detection of lymph node metastasis with Ir-PVP. ( a ) Optical images of ICR mice bearing 4T1 tumours in the paws show the hypoxic signals in the lymph nodes due to cancer cells metastasized to the nodes. Ir-PVP was administered through footpad injection in the right paw. The black arrows point to the area with lymph node metastases and the white arrows point to the primary tumour in the paw. ( b ) Bright and luminescent image of metastatic lymph node (left) and normal lymph node (right) 2 h after footpad injection of Ir-PVP in the right paw. ( c , d ) Haematoxylin and eosin-stained slices (× 200) of primary tumour ( c ) and lymph node metastases ( d ). ( e , f ) Frozen sections of the primary tumour ( e ) and lymph node with metastasis ( f ) were stained with HIF-1α antibody (green fluorescence). ( g , h ) Frozen sections of the primary tumour ( g ) and lymph node with metastasis ( h ) were stained with pimonidazole antibody (red fluorescence). Full size image Detection limit and tracking cancer cell proliferation in vivo To further evaluate the sensitivity of the Ir-PVP in detecting viable cancer cells in vivo , we continuously imaged the mice that were subcutaneously implanted with a small number of cancer cells while monitoring the cancer cell proliferation in vivo using Ir-PVP. After Ir-PVP was i.v. injected via the mouse tail vein (40 mg kg −1 ), different numbers of live H22 cells were injected subcutaneously into the armpit. Mice were imaged at selected time points from 1 to 96 h after injection. As shown in Fig. 7a , after the injection of 10 6 –10 7 H22 cells, a significant phosphorescence signal was detected in the cell-injected region at 1 h. The signal was detected in the region at 2 h after 10 5 cells were injected. When 10 4 and 10 3 cells were injected, the signal was detected at 6 and 24 h, respectively. No signal was detected when the injected cells were reduced to 10 2 or PBS was injected as the control. When photon counts in the cell-injected region were measured for the different amount of H22 cells injected, a positive correlation between the increase of signal intensity and the increased number of injected cells was observed at each time point ( Fig. 7b ). At 24 h post injection, the signal intensity of 10 3 H22 cells was 3.7-fold stronger than that of PBS control ( P <0.05), while there was no significant difference between the signal intensities of 10 2 H22 cells and the PBS control. 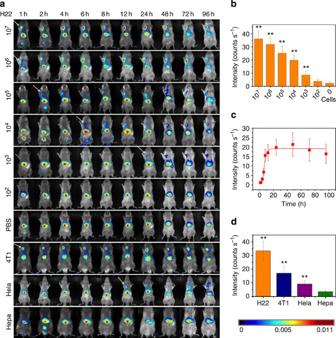Figure 7: Cancer cell detection limit and sensitivity of Ir-PVPin vivo. (a) Optical images of mice subcutaneously injected with different numbers of H22 cells (that is, 107, 106, 105, 104, 103and 102cells in 200 μl PBS), 4T1 cells (106in 200 μl PBS), HeLa cells (106in 200 μl PBS) and murine hepatocytes (Hepa, 106in 200 μl PBS). Cancer cells were implanted in the armpit, while Ir-PVP was injected via tail vein. The mice injected with PBS in the armpit were used as control. (b) The photon counts detected per second in the H22 cell-injected regions with different cell numbers (107, 106, 105, 104, 103, 102and 0) at 24 h post injection. The results are represented as the mean±s.d. (n=5). **P<0.01, in comparison of the signal intensities in the H22 cell-injected regions (102–107cells) and PBS-injected region (0 cells) using a one-way ANOVA. (c) The photon counts detected per second in the H22 cell-injected region at different time points after injection of 104H22 cells. (d) The photon counts detected per second in the cell-injected regions with different types of cells (H22, 4T1, HeLa and Hepa) at the same cell number (106) at 12 h post injection. The results are presented as the mean±s.d. (n=5). **P<0.01, in comparison between the signal intensities in the cancer cell-injected regions (H22, 4T1 and HeLa) and Hepa cell-injected region using ANOVA. Figure 7c shows the time-dependent signal intensity profile in the region with 10 4 H22 cells injected. In the first 12-h post injection, the signal intensity increased sharply over time. At 6 h post injection, the signal was sixfold stronger than the initial baseline and detectable by whole-body imaging. After 12 h post injection, the signal intensity increased to 20-fold stronger than the baseline. Thus, Ir-PVP exhibits the sensitivity of detecting more than 10 3 live H22 cells and their proliferation before these subcutaneously injected cells develop into mature tumours. Figure 7: Cancer cell detection limit and sensitivity of Ir-PVP in vivo . ( a ) Optical images of mice subcutaneously injected with different numbers of H22 cells (that is, 10 7 , 10 6 , 10 5 , 10 4 , 10 3 and 10 2 cells in 200 μl PBS), 4T1 cells (10 6 in 200 μl PBS), HeLa cells (10 6 in 200 μl PBS) and murine hepatocytes (Hepa, 10 6 in 200 μl PBS). Cancer cells were implanted in the armpit, while Ir-PVP was injected via tail vein. The mice injected with PBS in the armpit were used as control. ( b ) The photon counts detected per second in the H22 cell-injected regions with different cell numbers (10 7 , 10 6 , 10 5 , 10 4 , 10 3 , 10 2 and 0) at 24 h post injection. The results are represented as the mean±s.d. ( n =5). ** P <0.01, in comparison of the signal intensities in the H22 cell-injected regions (10 2 –10 7 cells) and PBS-injected region (0 cells) using a one-way ANOVA. ( c ) The photon counts detected per second in the H22 cell-injected region at different time points after injection of 10 4 H22 cells. ( d ) The photon counts detected per second in the cell-injected regions with different types of cells (H22, 4T1, HeLa and Hepa) at the same cell number (10 6 ) at 12 h post injection. The results are presented as the mean±s.d. ( n =5). ** P <0.01, in comparison between the signal intensities in the cancer cell-injected regions (H22, 4T1 and HeLa) and Hepa cell-injected region using ANOVA. Full size image Similar experiments were carried out with 4T1 and HeLa cells to examine the probe response to the oxygen consumption of the cancer cells. As shown in Fig. 7a , both subcutaneously injected 4T1 and HeLa cells (10 6 ) were detectable within 12 h post injection using Ir-PVP. However, no signal was detected when 10 6 murine hepatocytes, non-cancerous normal cells, were injected at any time, even 96 h after injection. Figure 7d shows the photon counts measured at 12 h post injection in the regions injected with 10 6 of H22, 4T1, HeLa and murine hepatocytes. The averaged signal intensities of H22, 4T1 and HeLa were nine-, five- and threefold, respectively, stronger than that of hepatocytes, indicating that the Ir-PVP probe is more specific to cancer cells rather than normal cells. When the rotenone (mitochondrial respiratory chain inhibitor) or oligomycin A (mitochondrial ATP-synthase inhibitor) was used to inhibit the oxygen consumption of cancer cells, it was found that the signal from the Ir-PVP probe decreased accordingly in the H22 cell-injected region after the treatment with the inhibitors ( Fig. 8a–d ). Rotenone and oligomycin A led to 2.5- and 2.3-fold of signal decrease, respectively. On the other hand, treatment with FCCP (carbonyl cyanide-4-(trifluoromethoxy)phenylhydrazone, an uncoupling agent) or ryanodine (an agent that causes cell deoxygenation via a calcium-mediated increase in metabolic rate), both of which promote the oxygen consumption of cancer cells [35] resulted in the signal increase ( Fig. 8e–h ). The signal increased by 1.9- and 1.8-fold for FCCP and ryanodine, respectively. These results not only provide additional evidence on that the detection of cancer cells by the probe is highly related to oxygen consumption of cancer cells, but also suggest potential applications of the probe in monitoring tumour development and treatment responses from the hypoxia-targeted therapeutics. 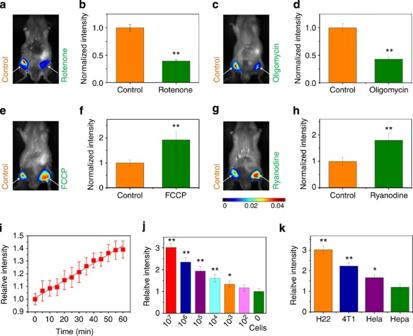Figure 8: Probe responses to the change of cancer cell oxygen consumption on drug treatments. (a–h) Luminescence images of ICR mice subcutaneously injected with 106H22 cells treated with rotenone (a), oligomycin A (c), FCCP (e) or ryanodine (g) in the right rear thigh muscle and 106untreated H22 cells in the left rear thigh muscle. Histogram showing the quantification of the signal intensities detected 1 h after the injection of 106H22 cells treated with rotenone (b), oligomycin A (d), FCCP (f) or ryanodine (h) and 106untreated H22 cells. The result represents the mean±s.d. (n=5). **P<0.01, in comparison between treated cells and untreated ones using a two-sample Student’st-test. (i) Monitoring the increase of the phosphorescence intensity of H22 cell suspension (107cells) incubated with Ir-PVP over time of 60 min. (j) Relative phosphorescence intensities of H22 cell suspensions with different cell numbers (107, 106, 105, 104, 103and 102) after incubation with Ir-PVP (0.1 mg ml−1) for 1 h. The pure incubation medium was used as control. The results represent the mean±s.d. (n=5). *P<0.05 and **P<0.01, in comparison between the H22 cell suspension and the blank control by a one-way ANOVA. (k) Comparison between the relative phosphorescence intensities of H22, 4T1, HeLa and murine hepatocytes (Hepa) cell suspension with the same cell number (107cells) after incubation with Ir-PVP (0.1 mg ml−1) for 1 h. The result was presented as the mean±s.d. (n=5). *P<0.05 and **P<0.01, in comparison between the intensities of cancer cell suspension (H22, 4T1 and HeLa) and Hepa cell suspension using ANOVA. Figure 8: Probe responses to the change of cancer cell oxygen consumption on drug treatments. ( a–h ) Luminescence images of ICR mice subcutaneously injected with 10 6 H22 cells treated with rotenone ( a ), oligomycin A ( c ), FCCP ( e ) or ryanodine ( g ) in the right rear thigh muscle and 10 6 untreated H22 cells in the left rear thigh muscle. Histogram showing the quantification of the signal intensities detected 1 h after the injection of 10 6 H22 cells treated with rotenone ( b ), oligomycin A ( d ), FCCP ( f ) or ryanodine ( h ) and 10 6 untreated H22 cells. The result represents the mean±s.d. ( n =5). ** P <0.01, in comparison between treated cells and untreated ones using a two-sample Student’s t -test. ( i ) Monitoring the increase of the phosphorescence intensity of H22 cell suspension (10 7 cells) incubated with Ir-PVP over time of 60 min. ( j ) Relative phosphorescence intensities of H22 cell suspensions with different cell numbers (10 7 , 10 6 , 10 5 , 10 4 , 10 3 and 10 2 ) after incubation with Ir-PVP (0.1 mg ml −1 ) for 1 h. The pure incubation medium was used as control. The results represent the mean±s.d. ( n =5). * P <0.05 and ** P <0.01, in comparison between the H22 cell suspension and the blank control by a one-way ANOVA. ( k ) Comparison between the relative phosphorescence intensities of H22, 4T1, HeLa and murine hepatocytes (Hepa) cell suspension with the same cell number (10 7 cells) after incubation with Ir-PVP (0.1 mg ml −1 ) for 1 h. The result was presented as the mean±s.d. ( n =5). * P <0.05 and ** P <0.01, in comparison between the intensities of cancer cell suspension (H22, 4T1 and HeLa) and Hepa cell suspension using ANOVA. Full size image To further verify that the probe signal is oxygen consumption dependent, cells were incubated with Ir-PVP in vitro , while the phosphorescence intensities of the probe were measured over time. As shown in Fig. 8i , a significant increase of phosphorescence intensity was detected from the suspension of 10 7 H22 cells incubated with Ir-PVP over time of 60 min, which is ascribed to the rapid oxygen consumption by the live H22 cells. The relative phosphorescence intensities of Ir-PVP in H22 cell suspensions, using pure incubation medium as a blank control, decreased as the cell number decreases (10 7 , 10 6 , 10 5 , 10 4 , 10 3 and 10 2 ; Fig. 8j ). At the cell number of 10 7 , the relative intensity was 3.0±0.2 ( P <0.01), while the intensity was 1.3±0.1 ( P <0.05) when the cell number decreased to 10 3 . Comparing different cells at the same cell number (10 7 ), probe concentration (0.1 mg ml −1 ) and incubation time (1 h), the signal intensities of probe in H22, 4T1, HeLa and murine hepatocytes decreased in order ( Fig. 8k ), indicating the trend of their decreased oxygen demand and oxygen consumption rate [36] . Taking together the results from the in vitro and in vivo experiments, we believe that the probe signal is hypoxia specific and closely correlated with the level of oxygen consumption of cancer cells with excellent sensitivity and detection limit. The current work reported the development of a hypoxia-specific NIR phosphorescent probe, Ir-PVP, for the sensitive detection of cancer cells and characterization of tumour hypoxia microenvironment in vivo . The signal from the probe is strongly correlated to the tissue oxygenation and oxygen consumption with minimal or no background signal from normal tissues. Compared with other molecular imaging probes, for instance, nitroimidazole [12] , Cu-diacetyl-bis( N -methylthiosemicarbazone) [37] and 18 F-Fluorodeoxyglucose [38] , which were previously used for direct or indirect detection of tumour hypoxia, Ir-PVP offers advantages of high specificity and high sensitivity to hypoxia with low non-specific signals. Hypoxia is an important characteristic of most advanced solid tumours [39] and hypoxic microenvironment plays an important role in tumour recurrence, metastasis and drug resistance. Hypoxic conditions are closely associated with the many events and pathways of tumour initiation and progression while presenting barriers to cancer therapies. The reported hypoxia-specific probe may provide a new approach for the early detection of cancer and characterization of cancer phenotypes based on their oxygen consumption and demand and their tendency to develop a hypo0xic tumour environment. As personalized and targeted treatments continue to be developed and available for patients, it is important to have non-invasive hypoxia imaging capability to assess the disruption of the tumour microenvironment and treatment responses. Determining the presence or absence of lymph node metastasis is crucial to the pathologic staging and prognostication of many lethal cancers [40] , [41] . Thus, a non-invasive method for the accurate assessment of lymph node involvement is highly necessary in the clinical management of cancer patients. To the best of our knowledge, Ir-PVP is the first hypoxia-sensitive optical probe that has been successfully applied for the detection of lymph node metastasis. The further translational development would enable Ir-PVP potentially to be used to detect lymph node metastasis non-invasively, either pre- or intraoperatively, based on the hypoxic condition created by cancer cells. In summary, a water-soluble, biocompatible and hypoxia-specific NIR-emitting probe, Ir-PVP, was developed for the non-invasive and sensitive imaging of hypoxia. With the reported probe, solid tumours and cancer cells metastasized to the lymph nodes can be detected with high sensitivity and low non-specific signal, based on the high oxygen consumption level in cancer cells. Furthermore, the proliferation of cancer cells can be also readily monitored with the reported imaging probe and NIR imaging before the formation of the solid tumour. Further, the probe can be readily modified for ratiometric measurement, allowing for the quantitative evaluation of the hypoxia level in cells and tumours. It is believed that Ir-PVP provides a hypoxia-specific imaging tool for detecting the presence of cancer cells early and assessing tumour microenvironment in vivo using the NIR optical imaging method. Synthesis of Ir-PVP Detailed description of the synthesis of Ir-PVP can be found in the Supplementary Methods . Ir-PVP was characterized by 1 H and 13 C NMR spectroscopy, gel permeation chromatography, Fourier transform infrared spectra and ultraviolet–visible spectra. Characterization data of Ir-PVP: 1 H NMR (600 MHz, CDCl 3 ): δ 9.27 (d, J=8.3 Hz, 1H, 1-H phenanthridine), 9.06 (d, J=8.2 Hz, 1H, 1-H phenanthridine), 8.80 (d, J=8.3 Hz, 1H, 4-H phenanthridine), 8.65 (d, J=8.4 Hz, 1H, 4-H phenanthridine), 8.56 (d, J=8.2 Hz, 1H, 4-H benzo[b]thiophene), 8.19 (d, J=8.2 Hz, 1H, 4-H benzo[b]thiophene), 8.04–7.99 (m, 2H, 2, 6-H PhCO), 7.94 (t, J=7.8 Hz, 2H, 3-H phenanthridine), 7.86 (t, J=7.7 Hz, 1H, 2-H phenanthridine), 7.71 (d, J=8.0 Hz, 1H, 7-H phenanthridine), 7.58 (d, J=8.0 Hz, 1H, 7-H phenanthridine), 7.52 (t, J=7.7 Hz, 1H, 2-H phenanthridine), 7.33 (m, 4H, 7-H benzo[b]thiophene, 9-H phenanthridine), 7.09–7.04 (m, 2H, 3, 5-H PhCO), 6.91 (m, 2H, 8-H phenanthridine), 6.55 (t, J=7.8 Hz, 2H, 6-H benzo[b]thiophene), 6.42 (d, J=8.3 Hz, 1H, 10-H phenanthridine), 6.33 (t, J=7.7 Hz, 1H, 5-H benzo[b]thiophene), 6.30 (t, J=7.8 Hz, 1H, 5-H benzo[b]thiophene), 6.06 (d, J=8.1 Hz, 1H, 10-H phenanthridine), 5.18 (s, 1H, COCH), 3.72 (m, broad, 125H, PVP NCH), 3.21 (m, broad, 248H, PVP NCH 2 ), 2.36–1.41 (m, broad, 741H, PVP CHCH 2 , COCH 2 , NCH 2 CH 2 ); 13 C NMR (150 MHz, CDCl 3 ): δ 188.2 (C), 175.4 (C, PVP), 161.2 (C), 132.3 (C), 131.9 (CH), 131.6 (CH), 129.3 (CH), 129.1 (C), 128.4 (CH), 127.7 (CH), 127.3 (CH), 126.6 (CH), 125.9 (CH), 125.2 (CH), 124.7 (CH), 123.9 (CH), 122.4 (CH), 121.7 (C), 112.9 (CH), 95.2 (CH), 44.9 (CH, PVP), 42.1 (CH 2 , PVP), 35.5 (CH 2 , PVP), 31.5 (CH 2 , PVP), 18.3 (CH 2 , PVP); M n (NMR)=14,100 Da, M n (gel permeation chromatography)=13,000 Da, PDI=1.50; IR: 1,652 cm −1 ; ultaviolet/visible: λ max 530, 560 nm. Cell culture and cellular uptake of the probes Two cell lines, the human neuroblastoma SH-SY5Y cell line and the murine hepatic cancer H22 cell line, were used. The cells were cultured in DMEM (Dulbecco’s modified Eagle’s medium) supplemented with 10% fetal bovine serum at 37 °C under 5% CO 2 . The probe was added to the media at a final concentration of 0.2 mg ml −1 . The cells were incubated for 2 h and washed three times with PBS (pH=7.4). After that, the cells were further incubated at three oxygen concentrations (21, 10 and 0%) for another 1 h at 37 °C. The cells were observed with confocal laser scanning microscopy (CLSM, Zeiss LSM-710 microscope, Germany). For Ir-PVP, the cells were excited at 543 nm and the signal was received at 650–750 nm. For Ir-PVP-RhB, cells were excited at 514 nm and the signal was received at two channels, 540–610 nm and 670–750 nm. Anaero Pack-Anaero and Anaero Pack-Micro Aero (Mitsubishi Gas Chemical Co. Inc., Japan) were used to provide cell culture environments with oxygen concentrations of 0 and 10%. Hypoxia imaging of MCs A layer of poly-(2-hydroxyethyl methacrylate) (poly-HEMA) film was coated on the bottom of tissue culture flasks (T25). Poly-HEMA (450 mg) was dissolved in 95% ethanol (30 ml) and the mixture was shaken slowly for 24 h at 37 °C. When the polymer was completely dissolved, 4 ml of the mixture was pipetted into a tissue culture flask. The flask was then allowed to dry for 48 h at 37 °C. To ensure sterility, poly-HEMA-coated flasks were exposed to ultraviolet light for 2 h before use. SH-SY5Y cells in monolayer culture were trypsinized to give a single-cell suspension and the cell number was counted using a haemocytometer. Cells (5 × 10 5 ) were added to 5 ml of fresh DMEM medium in each poly-HEMA-coated flask. Cells were incubated at 37 °C in humidified atmosphere with 5% CO2 and the culture medium was replaced every other day. The SH-SY5Y MCs with diameters about 250–350 μm were harvested after ~7 days of growth [42] . For each experiment, ~20 spheroids were handpicked with a Pasteur pipette and transferred to a 5-ml eppendorf tube. The probe was added to the spheroids suspension at a final concentration of 0.2 mg ml −1 and co-cultured for 4–24 h at 37 °C. Then the media were removed. The MCs were washed with PBS (pH=7.4) and observed with CLSM (Zeiss LSM-710 microscope, Germany). Tumour model and hypoxia imaging All animal experiments were performed in compliance with the guidelines set by the Animal Care Committee at Drum Tower Hospital. To establish a subcutaneously implanted H22 tumour model, H22 cells (5 × 10 6 cells dispersed in 200 μl PBS) were injected subcutaneously into the armpit of 10 ICR mice (aged 6–8 weeks, 22–26 g). Tumour growth was monitored until it reached the size of 5–10 mm in diameter before it was ready for the experiments. Then, 200 μl Ir-PVP (5 mg ml −1 in PBS) was injected into the mice via the tail vein. Mice were then imaged at 1, 2, 4, 8, 24, 48, 72, 96, 120 h post injection using the Maestro EX fluorescence imaging system (Cambridge Research & Instrumentation, CRi, USA). At 120 h post injection, mice were killed by cervical dislocation and the major organs were harvested and immediately imaged. The entire procedure from mouse killing to the end of imaging was completed within 5 min (ref. 43 ). Detection of lymph node metastasis 4T1 cells (10 6 cells in 40 μl PBS) were injected into the right rear paw of five BALB/c nude mice. Four weeks later, the right inguinal lymph node swelled up, indicating the presence of metastases. Ir-PVP (10 μl, 5 mg ml −1 in PBS) was injected into the right rear paw and gently massaged for 5 min and then the mice were imaged at predetermined time intervals. After that, the primary tumour and the right inguinal lymph node were dissected and assessed by haematoxylin and eosin staining and immunofluorescence staining. Detection of cancer cells in vivo Ir-PVP (200 μl, 5 mg ml −1 in PBS) was injected into ICR mice (6–8 weeks, 22–26 g) via the tail vein. Mice ( N =5 per group) were then subcutaneously injected with 200 μl of H22 cell suspensions with different concentrations (5 × 10 7 , 5 × 10 6 , 5 × 10 5 , 5 × 10 4 , 5 × 10 3 , 5 × 10 2 cells ml −1 in PBS) in the armpit. The mice subcutaneously injected with 200 μl PBS in the armpit were used as controls. Optical imaging experiments were performed at 1, 2, 4, 6, 8, 12, 24, 48, 72 and 96 h after the injection of H22 cells. Other cell lines, 4T1 and murine hepatocytes, were injected using the same procedure as that used for H22. For experiments with HeLa cells, BALB/c nude mice were used. Immunofluorescence staining Tumours were surgically excised 30 min after i.v. injection with pimonidazole hydrochloride (60 mg kg −1 ). Frozen sections of the tumours were prepared with OCT compound (Sakura Finetek). Primary antibodies used were as follows: anti-HIF-1α rabbit polyclonal antibody (diluted 150 times, Santa Cruz Inc.), anti-pimonidazole mouse monoclonal antibody conjugated to FITC (FITC-Mab1, diluted 250 times, Hypoxyprobe-1 Plus Kit, Hypoxyprobe Inc., Burlington). HIF-1α was detected with Alexa Flour 488-conjugated goat anti-rabbit secondary antibody diluted for 300 times. Pimonidazole was detected with Dylight-594 conjugated mouse anti-FITC secondary antibody (diluted 500 times, Jackson Immuno Research Laboratories, West Grove, PA). The images were captured with CLSM (Zeiss LSM-710 microscope). Statistical analysis Quantitative data were expressed as mean±s.d. Statistical comparisons were made by ANOVA and Student’s t -test. A P value <0.05 was considered statistically significant. How to cite this article: Zheng, X. et al . Hypoxia-specific ultrasensitive detection of tumours and cancer cells in vivo . Nat. Commun. 6:5834 doi: 10.1038/ncomms6834 (2015).